Symmetry protected Josephson supercurrents in three-dimensional topological insulators Coupling the surface state of a topological insulator to an s-wave superconductor is predicted to produce the long-sought Majorana quasiparticle excitations. However, superconductivity has not been measured in surface states when the bulk charge carriers are fully depleted, that is, in the true topological regime relevant for investigating Majorana modes. Here we report measurements of d.c. Josephson effects in topological insulator–superconductor junctions as the chemical potential is moved through the true topological regime characterized by the presence of only surface currents. We compare our results with three-dimensional quantum transport simulations, and determine the effects of bulk/surface mixing, disorder and magnetic field; in particular, we show that the supercurrent is largely carried by surface states, due to the inherent topology of the bands, and that it is robust against disorder. Our results thus clarify key open issues regarding the nature of supercurrents in topological insulators. Three-dimensional (3D) topological insulators (TIs), such as Bi 2 Se 3 and Bi 2 Te 3 , are characterized by the existence of a bulk-insulating energy gap, gapless Dirac surface states and a π -Berry’s phase [1] . For 3D TIs coupled to s-wave superconductors, the winding of the superconducting vortices can counteract the π -Berry’s phase, resulting in zero-energy Majorana fermions produced at the interface [2] , [3] , [4] , [5] . Such Majorana fermions may be topologically protected from decoherence, and could have a significant role in solid-state implementations of a quantum computer. A requisite step in the search for Majorana fermions is to understand the nature and origin of the supercurrent generated between superconducting contacts and a TI. Previous measurements of Bi 2 Se 3 - or Bi 2 Te 3 -superconductor junctions [6] , [7] , [8] , [9] have demonstrated that the supercurrent can be tuned by a gate voltage [8] and exhibits Josephson effects such as Fraunhofer patterns [6] , [9] ; it has also been argued that the supercurrent is carried by surface states, though the mechanism was not well understood [6] . Fundamental questions remain, particularly concerning the behaviour through the Dirac point and the effects of disorder. We approach these by measuring the supercurrent over a wide-range of gate voltages (chemical potentials)—through a clear ambipolar transport regime—and by comparing our results with full 3D quantum transport calculations that can include disorder. We find that the supercurrent is largely carried by surface states because of protected crystal symmetries, and is only suppressed when bulk/surface mixing is strong or at very low carrier densities. We further find that the supercurrent is not symmetric with respect to the conduction and valence bands, and that the Fraunhofer patterns are similar both within and outside of the topological regime. Approaching the topological regime The major obstacles in reaching the topological regime in transport experiments are high n-doping in as-grown TI materials and the further increase of n-doping during mechanical cleavage of crystals [10] , [11] , [12] , [13] . We implemented three strategies to reduce doping in thin exfoliated films, utilizing (1) Sb-doped TI materials, (2) chemical doping of the top surface and (3) a backgate. It has been previously reported that growing 3D TI materials with in-situ Ca or Sb dopants reduces n-doping [10] , [13] , [14] , [15] . Thus, we have grown (Bi x Sb 2− x )Se 3 crystals having x =1.33 (see Methods ). Angle-resolved photoemission spectroscopy (ARPES) confirms the topological spectra of the crystals (Fig. 2d). From Fig. 2d, it is evident that the bulk conduction band (BCB) is located at an energy E ~0.20 eV above the Dirac point and gapless linear surface states exist inside the bulk bandgap. The total surface carrier density at the bottom of the BCB is estimated to be k 2 /4 π × 2 (two surfaces of a device)~0.8 × 10 13 cm −2 , where k ~0.071 Å −1 was extracted at the bottom of the BCB from the ARPES data along the Γ–K line. Possible hexagonal warping of the Fermi surface could lead to few percent error in the carrier density near the bottom of the BCB [16] . Devices consisted of mechanically exfoliated ~10-nm-thick films on Si/SiO 2 substrates [10] , [11] , [12] (which are used as backgates) having Ti(2.5 nm)/Al(140 nm) contacts (see Methods ). We deposited the chemical dopant 2,3,5,6-tetrafluoro-7,7,8,8-tetracyanoquinodimethane (F4-TCNQ) on some devices, as shown schematically in Fig. 1a . F4-TCNQ has a strong electron affinity, and has been shown to effectively remove excess n-doping in Bi 2 Se 3 (ref. 12 ). A backgate voltage was then used to fully deplete the bulk charge carriers and tune the chemical potential through the Dirac point. It has been shown that once the bulk charge carriers are mostly depleted, the Fermi levels of the top and bottom surface states lock to each other and shift simultaneously, even with a single gate [12] . In this paper, we show experimental results from two devices, where ‘device 1’ has chemical doping and ‘device 2’ does not. It was possible to use a backgate to deplete bulk carriers in device 2 because of the low n-doping due to Sb; however, in this case a much larger backgate voltage was required to reach the Dirac point. All transport measurements were performed in a dilution refrigerator at the base temperature of T =16 mK. Each device was configured with both a Hall bar geometry and with closely spaced electrodes across which Josephson currents were measured, as shown in Fig. 1a and b . 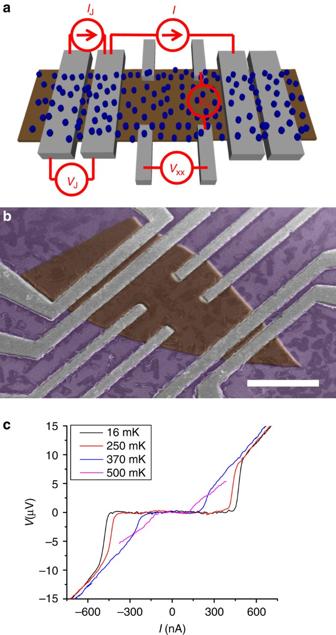Figure 1: Measurement configuration and supercurrent characterization (a) Device and measurement schematic and (b) scanning electron microscopy image of device 1. The blue dots inarepresent 2,3,5,6-tetrafluoro-7,7,8,8-tetracyanoquinodimethane (F4-TCNQ) molecules. The Hall measurement was performed in the Hall bar by applying currentIand measuring longitudinal (Vxx) and Hall (VH) voltages, while the Josephson effect was measured in the closely spaced junction by applying currentIJand measuring voltageVJ. The scale bar inbcorresponds to 1 μm. (c)I–Vcurves measured in device 2 atVg=0 for four different temperatures, showing typical supercurrent behaviour. Figure 1: Measurement configuration and supercurrent characterization ( a ) Device and measurement schematic and ( b ) scanning electron microscopy image of device 1. The blue dots in a represent 2,3,5,6-tetrafluoro-7,7,8,8-tetracyanoquinodimethane (F4-TCNQ) molecules. The Hall measurement was performed in the Hall bar by applying current I and measuring longitudinal ( V xx ) and Hall ( V H ) voltages, while the Josephson effect was measured in the closely spaced junction by applying current I J and measuring voltage V J . The scale bar in b corresponds to 1 μm. ( c ) I–V curves measured in device 2 at V g =0 for four different temperatures, showing typical supercurrent behaviour. 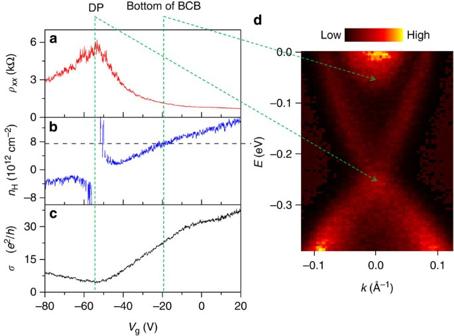Figure 2: Normal state characterization. (a) Longitudinal resistivityρxx, (b) Hall carrier densitynHand (c) longitudinal conductivityσxxfor device 1 as functions of backgate voltage. The maximum inρxx(min inσxx) and divergence ofnHindicate the location of the Dirac point (DP) and the presence of both carrier types. (d) ARPES data of the bulk crystal along theΓ–Kline, showing the expected Dirac cone band structure of the surface state. The Dirac point and the bottom of the bulk conductance band (BCB) are indicated by arrows. It is clear from ARPES and Hall data that the system passes through a true topological regime of only surface states. Full size image Hall measurements Figure 2 shows resistivity and Hall measurements for device 1 at T =16 mK and with B perpendicular =35 mT (to suppress superconductivity in the aluminium leads). We observe a peak in resistivity ρ xx (minimum in conductivity σ xx ) and a corresponding sign change in Hall carrier density n H near V g ~−55 V, which signal that the charge carriers change from electrons to holes as the chemical potential passes through the Dirac point. Figure 2 shows that the charge neutrality point seems to coincide with the minimum conductivity (or maximum resistivity) point. The negligible difference of residual densities of electrons and holes in the Hall measurement also implies that the charge neutrality and Dirac points are reached at nearly the same gate voltage [17] . By comparing the total surface carrier density at the bottom of the BCB calculated from ARPES measurements, n H= 0.8 × 10 13 cm −2 , to the n H versus V g measured in Fig. 2b , we find that the bottom of the BCB occurs near V g =−18 V (with a few volt uncertainty due to possible hexagonal warping). This indicates that V g <−18 V is the topological regime, where only surface states are occupied, while V g >−18 V is the regime where both surface and bulk states are populated. Figure 2: Normal state characterization. ( a ) Longitudinal resistivity ρ xx , ( b ) Hall carrier density n H and ( c ) longitudinal conductivity σ xx for device 1 as functions of backgate voltage. The maximum in ρ xx (min in σ xx ) and divergence of n H indicate the location of the Dirac point (DP) and the presence of both carrier types. ( d ) ARPES data of the bulk crystal along the Γ–K line, showing the expected Dirac cone band structure of the surface state. The Dirac point and the bottom of the bulk conductance band (BCB) are indicated by arrows. It is clear from ARPES and Hall data that the system passes through a true topological regime of only surface states. Full size image Josephson effects We now turn to measurements of Josephson effects. Figure 1c shows I–V curves measured for device 2 at three different temperatures, for V g =0. The I–V curves exhibit zero-voltage regimes for currents less than the critical current I c . Above I c , a finite voltage is measured as the sample transitions to the normal regime. The critical current can also be modulated by V g : in Fig. 3b and d , we show two-dimensional plots of differential resistance d V/ d I versus current I versus V g , for devices 1 and 2, respectively. The purple regions where d V/ d I=0 indicate superconducting regions, and the boundary corresponds to I c for a given V g . 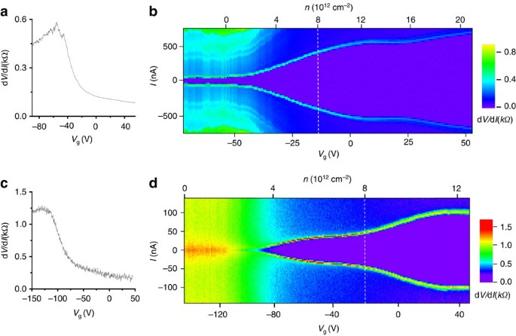Figure 3: Dependence of supercurrents on gate voltage. Differential resistance (dV/dI) versus gate voltage in the normal regime (B=35 mT) for (a) device 1 and (c) device 2, showing locations of Dirac points in the Josephson configuration. Two-dimensional plots of dV/dIversus gate voltageVgand currentIfor (b) device 1 and (d) device 2. The purple regions show the extent of the supercurrent, where dV/dI=0; the boundaries of these regions correspond toIc. The bottom of the bulk conduction band is labelled as white dashed lines inbandd. Figure 3a and c show the corresponding normal state d V/ d I versus V g for the two-terminal Josephson configuration (taken at B =35 mT). For device 1, the Dirac point is identified with the maximum resistance peak at V g ~−55 V, consistent with the Hall measurement shown in Fig. 2 ; the Dirac point for device 2 is near V g ~−140 V. Figure 3: Dependence of supercurrents on gate voltage. Differential resistance (d V/ d I ) versus gate voltage in the normal regime ( B =35 mT) for ( a ) device 1 and ( c ) device 2, showing locations of Dirac points in the Josephson configuration. Two-dimensional plots of d V/ d I versus gate voltage V g and current I for ( b ) device 1 and ( d ) device 2. The purple regions show the extent of the supercurrent, where d V/ d I =0; the boundaries of these regions correspond to I c . The bottom of the bulk conduction band is labelled as white dashed lines in b and d . Full size image It is now possible to compare the behaviour of the supercurrent in different transport regimes. Figure 3 shows that in both devices, the critical current decreases, non-monotonically, as the Dirac point is approached from the conduction band, and does not increase significantly in the valence band. Focusing first on device 1 ( Fig. 3b ), we note that the system does not seem to change behaviour at the position of the bottom of the BCB ( V g ~−18 V). Below the BCB , I c continues to decrease until it reaches the Dirac point, near which it saturates to a small but finite value. The finite I c near the Dirac point may be caused by residual densities in electron-hole puddles due to charged impurity potentials [12] , [18] , [19] , [20] . Surprisingly, the critical current does not increase in the hole region ( V g <−55 V); this may be related to asymmetric contact resistances [21] or to the lack of clear surface states in the valence band (as seen in Fig. 2d ). In device 2 ( Fig. 3d ), I c becomes zero at large negative gate voltages, even before the Dirac point is reached. In fact, d V/ d I exhibits a peak for V g <−100 V, the height of which increases with lower temperatures. The different behaviour of device 2 at low densities may be due to increased disorder or longer channel length [22] . We also examine a further hallmark of the Josephson effect, Fraunhofer behaviour, inside and outside of the topological regime. 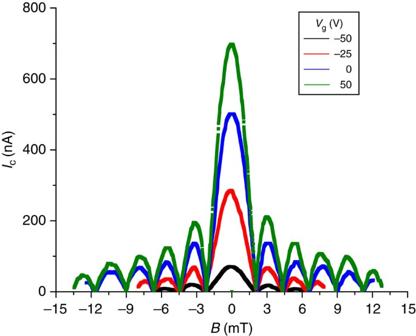Figure 4: Fraunhofer data. Critical supercurrentIcversus perpendicular magnetic fieldBatT=16 mK for device 1 at different gate voltages, showing clear Fraunhofer diffraction patterns. The minima occur at intervals ofФ/Ф0~0.23n, wherenis an integer; however, we plotIcversusBrather thanФ/Ф0because the short junction area may be ill-defined due to flux focusing26. Figure 4 shows a plot of measured I c as a function of magnetic field B in device 1 at different gate voltages. The resulting Fraunhofer patterns, the single-slit interference-like dependence of I c on B in a Josephson junction, demonstrate that the supercurrent through the junction originates from the Josephson effect. 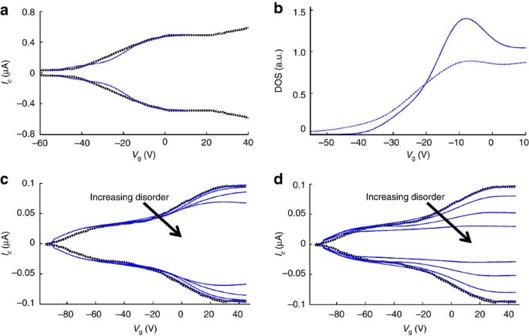Figure 5: Comparisons of experiment with 3D simulations that include disorder. (a) Dependence of critical currentIcon gate voltageVgfor a short channel junction (1:3 length to width ratio) (blue), overlayed with experimental results from device 1 (dashed black). (b) Surface (dashed blue) and bulk (solid blue) density of states (DOS) for the model topological insulator Hamiltonian, mapped toVgfor device 1. The bulk is gapped, with the first states appearing near −38 V (though the majority of bulk subbands appear above −20 V). The peak in the bulk DOS nearVg~ −10 V is not consistent with the monotonicity of the bulk DOS seen in the angle-resolved photoemission spectroscopy data; however,Fig. 4ashows that the bulk DOS does not have a significant role in transport within the junction, and thus the model can capture the salient transport physics. The effect of (c) bulk disorder and (d) surface and bulk disorder onIcin a long-channel junction (2:1 length to width ratio), for δ-impurity strengths equal to 0, 0.2, 0.5 and 1.0 times the bulk bandgap energy. For this device, bulk states become dominant at approximately −20 V (the DOS is similar to that in 5b, but the gate voltage axis would range from −95 to 45 V due to the disparity in backgate capacitance between devices). Inc, the supercurrent only decreases appreciably when the bulk disorder potential is large enough to begin hybridizing bulk and surface bands. Including surface disorder, as ind, causes the supercurrent to degrade immediately, signifying that supercurrent flows primarily through the surface band. Experimental results from device 2 are overlayed on both plots (dashed black). Figure 5 shows that while the amplitude of I c changes with V g , the period of oscillation of I c with B does not, for measurements both within and outside the topological regime. Figure 4: Fraunhofer data. Critical supercurrent I c versus perpendicular magnetic field B at T =16 mK for device 1 at different gate voltages, showing clear Fraunhofer diffraction patterns. The minima occur at intervals of Ф/Ф 0 ~0.23 n , where n is an integer; however, we plot I c versus B rather than Ф/Ф 0 because the short junction area may be ill-defined due to flux focusing [26] . Full size image Figure 5: Comparisons of experiment with 3D simulations that include disorder. ( a ) Dependence of critical current I c on gate voltage V g for a short channel junction (1:3 length to width ratio) (blue), overlayed with experimental results from device 1 (dashed black). ( b ) Surface (dashed blue) and bulk (solid blue) density of states (DOS) for the model topological insulator Hamiltonian, mapped to V g for device 1. The bulk is gapped, with the first states appearing near −38 V (though the majority of bulk subbands appear above −20 V). The peak in the bulk DOS near V g ~ −10 V is not consistent with the monotonicity of the bulk DOS seen in the angle-resolved photoemission spectroscopy data; however, Fig. 4a shows that the bulk DOS does not have a significant role in transport within the junction, and thus the model can capture the salient transport physics. The effect of ( c ) bulk disorder and ( d ) surface and bulk disorder on I c in a long-channel junction (2:1 length to width ratio), for δ-impurity strengths equal to 0, 0.2, 0.5 and 1.0 times the bulk bandgap energy. For this device, bulk states become dominant at approximately −20 V (the DOS is similar to that in 5b, but the gate voltage axis would range from −95 to 45 V due to the disparity in backgate capacitance between devices). In c , the supercurrent only decreases appreciably when the bulk disorder potential is large enough to begin hybridizing bulk and surface bands. Including surface disorder, as in d , causes the supercurrent to degrade immediately, signifying that supercurrent flows primarily through the surface band. Experimental results from device 2 are overlayed on both plots (dashed black). Full size image To explain the unique features observed in I c versus V g , we compare the experimental data to transport simulations of a model that couples superconducting contacts to a 3D tight-binding Dirac Hamiltonian with an inverted mass gap; this creates a topologically non-trivial Josephson junction that retains the geometry of the samples ( Supplementary Notes 1 and 2 ). Supercurrents and density of states (DOS) profiles are calculated in the non-equilibrium Green function formalism [23] . Figure 5a shows results for a geometry similar to device 1 overlayed with the measurements; there is excellent correspondence between simulations and experiment. To understand the I c versus V g behaviour, we plot the bulk and surface DOS for device 1 in Fig. 5b . Although the model we employ yields residual bulk DOS at V g <−20 V, brought about by a single bulk subband beginning at V g =−38 V (set by computational constraints on the Hamiltonian parameters, see Supplementary Note 2 ), the majority of bulk subbands first appear near V g =−20 V. As we show below, the bulk is largely inert, and I c is not dependent on the BCB minimum, so that numerical and experimental results remain compatible. We note that above the Dirac point, I c closely follows the surface DOS throughout the entire energy range, which explains the non-monotonic behaviour of I c . The fact that the supercurrent closely matches the surface DOS profile implies that the Josephson current is predominantly carried by the topological surface band, independent of bulk characteristics. Figure 5c shows simulations for a geometry similar to device 2 overlayed with the measurements; again, the simulations match the experiments. The supercurrent has a shape similar to that of device 1, but an insulating regime arises near the Dirac point. This may suggest that for longer junctions the channel becomes insulating above a critical resistance [22] . To further understand the surface-dominated supercurrent, we added δ-function impurities of increasing strength (see Supplementary Note 3 ) to bulk and/or surface regions in the long-channel model (2:1 length to width ratio) to determine the effect of degraded bulk and surface mobility on critical supercurrent. For the model, the bulk and surface are both considered to have mean free paths much longer than the sample size. The effect of disorder localized in the bulk versus disorder in both surface and bulk is shown in Fig. 5c and d , respectively. Decreased bulk mobility (due to disorder) has little effect on I c until the disorder strength becomes large enough to hybridize the surface band with the bulk, that is, when the impurity strength is comparable to the bandgap energy. Disorder applied equally to bulk and surface states, in contrast, results in a continuous degradation of current as disorder is increased. These simulations strongly suggest that the large majority of supercurrent is carried along the surface of the TI, and that this occurs because of crystal symmetries rather than a discrepancy in bulk and surface mobilities. This is in stark contrast to normal state transport simulations for Bi 2 Se 3 , which have shown that when the chemical potential is pushed out of the purely topological regime, current flows primarily through the bulk due to the onset of many additional available states [24] . We find that the supercurrent only degrades if the surface is encumbered with elastic scattering centres, or if bulk disorder is so large that surface-bulk band hybridization occurs. Crystal growth The crystals of Bi 1.33 Sb 0.67 Se 3 were grown by using a modified floating zone method in which the melting zone is Se-rich BiSbSe. The materials of high purity 99.9999% Bi, Sb and Se were premelted and loaded into a 10-mm diameter quartz tube. The crystal growth velocity in the quartz tube is 0.5 mm per hour. ARPES The ARPES experiments were carried out at the National Synchrotron Light Source, using the VUV undulator beamline U13UB, which is based on a 3-m normal incidence monochromator. The photon energy used in the study was 20.5 eV. The electron analyzer was a Scienta SES-2002, which uses a two-dimensional micro-channel plate as a detector that collects simultaneously a wide energy window and a wide angular window (~14°) of excited photoelectrons. The combined energy resolution was around 8 meV, while the angular resolution was better than ~0.15°, translating into a momentum resolution of~0.005 Å −1 at 20.5 eV photon energy. Samples were mounted on a liquid He cryostat and cleaved in situ and measured at ~15 K in the ultrahigh vacuum chamber with the base pressure 3 × 10 −9 Pa. Device fabrication and measurement We mechanically exfoliated thin films from bulk (Bi 1.33 Sb 0.67 )Se 3 crystals on 300 nm SiO 2 /highly n-doped Si substrates by the ‘scotch tape method’ [25] ; films of thickness ~10 nm were found by optical microscope and atomic force microscopy [10] , [11] , [12] . Device 1 has a thickness of 14 nm and dimensions L ~0.1 μm and W ~1.4 μm, whereas device 2 has a thickness of 12 nm and dimensions L ~0.5 μm and W ~2.5 μm. Subsequently, electron beam lithography was performed to define a Hall bar and closely spaced junctions in a device. Brief surface cleaning with ion milling and Ti(2.5 nm)/Al(140 nm) deposition were performed at a base pressure~1 × 10 −9 Torr with sample substrates cooled to T ~77 K. Immediately after lift-off, device 2 was wire-bonded and cooled down in a commercial dilution refrigerator. About 8 nm of F4-TCNQ (Sigma-Aldrich) was deposited on device 1 before wire-bonding and cool-down. We observed 2–3 times higher backgate capacitance ( n=C g V g /e , where C g =20–30 nF cm −2 ) in device 1 (with chemical dopants), compared with C g ~11 nF cm −2 in device 2 (with no chemical dopants). Similar values of enhanced backgate capacitance at low temperature in thin Bi 2 Se 3 devices doped with polymer electrolyte were reported previously, [12] however the origin is not well understood. How to cite this article: Cho, S. et al . Symmetry protected Josephson supercurrents in three-dimensional topological insulators. Nat. Commun. 4:1689 doi: 10.1038/ncomms2701 (2013).